Single-molecule detection of dihydroazulene photo-thermal reaction using break junction technique Charge transport by tunnelling is one of the most ubiquitous elementary processes in nature. Small structural changes in a molecular junction can lead to significant difference in the single-molecule electronic properties, offering a tremendous opportunity to examine a reaction on the single-molecule scale by monitoring the conductance changes. Here, we explore the potential of the single-molecule break junction technique in the detection of photo-thermal reaction processes of a photochromic dihydroazulene/vinylheptafulvene system. Statistical analysis of the break junction experiments provides a quantitative approach for probing the reaction kinetics and reversibility, including the occurrence of isomerization during the reaction. The product ratios observed when switching the system in the junction does not follow those observed in solution studies (both experiment and theory), suggesting that the junction environment was perturbing the process significantly. This study opens the possibility of using nano-structured environments like molecular junctions to tailor product ratios in chemical reactions. The switching of photochromic molecules is accompanied by changes in electronic, structural and/or chemical properties, making photoswitches versatile building blocks for potential applications in materials science, electronics and biotechnology [1] , [2] , [3] . Progress in this area requires detailed understanding of these molecules and various analytical techniques have been used to analyse the photoreaction process, such as ultraviolet–visible (UV–Vis) spectroscopy, fluorescence spectroscopy [4] , [5] and Raman spectroscopy [6] , [7] . As a potential analytical tool, the single-molecule break junction technique has been employed to study the conductance–structure correlation of a large range of molecular components in the past years [8] , [9] , [10] , [11] , [12] , [13] , [14] . More importantly, the break-junction techniques could also provide a means to statistically quantify the photo-reaction kinetics of a single-molecule device connected between two electrodes, which may offer some new understanding beyond measuring an ensemble of molecules as in other spectroscopies. We became interested in exploring the dihydroazulene ( dha )/vinylheptafulvene ( vhf ) system [15] , [16] as previous studies have shown light-controlled conductance switching of dha derivatives in a silver nanogap fabricated using sublimable molecules and also bias-induced switching for a junction operating in the Coulomb blockade regime [17] , [18] . Fabrication of junctions by sublimation puts some constraints on the molecules that can be studied in regard to molecular weight and stability. The break-junction technique employs a solution of the molecules and it has allowed us to achieve charge transport properties of larger dha molecules by incorporating anchoring groups (−SAc) at each end of the molecule to control the anchoring configuration. We employ the mechanically controllable break junction (MCBJ) technique to detect the photo-thermal reaction processes of a tailor-made photochromic dha / vhf system. Three distinguishable conductance states are observed experimentally, while reversible and distinct changing of the single molecular conductance is observed between two of the states. Benefiting from the well-distinguished conductance states, the reaction kinetics and reversibility could be studied via statistical analysis of the conductance–distance traces, and it is found that the reaction in the junction does not follow those observed in solution, which agrees well with the energy calculation. Density functional transport calculations reproduce the relative conductance of these molecular states and identify a changing destructive interference effect as being responsible for the large span in conductance. Single-molecule conductance measurement We measured the single-molecule conductance of the target molecules using the MCBJ technique under ambient conditions [19] , [20] . The MCBJ measurements proceeded as follows: the contacted point of the two electrodes was repeatedly broken and reformed in the solution containing 0.2 mM target molecule under the control of piezo-stack movement. During the breaking process, the anchoring groups (thioacetates) can contact the surface of gold electrodes via Au–S bond and bridge the molecule between the separated electrodes to form the Au-molecule-Au junction. Under a fixed bias (100 mV), the current through the junction was recorded and is used for the further analysis. 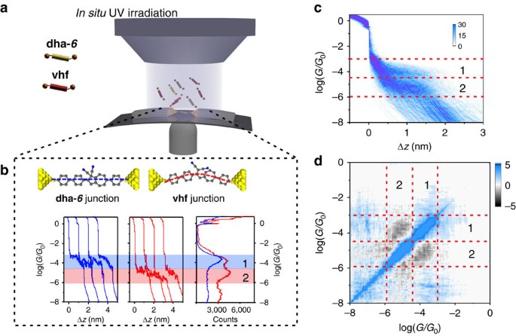Figure 1: Single-molecule conductance measurements. (a) Schematic of the mechanically controllable break junction (MCBJ) measurements during the photo-conversion of dihydroazulene under thein situultraviolet (UV) irradiation. The solution contains dihydroazulene (dha-6) and vinylheptafulvene (vhf). (b) Typical individual conductance–distance traces recorded in break junction measurements; blue for thedha-6junction and red for thevhfjunction. The applied bias potential is 100 mV. (c) 2D conductance–displacement histogram constructed from 1,000 conductance–distance traces, the conductance region 10−3.0∼10−4.5G0is defined as region 1, and the conductance region 10−4.5∼10−6.0G0is defined as region 2. Linear scaling is applied for the colour bar. (d) 2D covariance histogram constructed from 1,000 conductance–distance traces. Figure 1b shows the typical conductance traces plotted on a logarithmic scale. The plateaus with a conductance value below G 0 (conductance quantum) are assigned to molecular junctions. Hundreds to thousands of conductance traces are used to construct the one-dimensional (1D) histograms and two-dimensional (2D) histograms. Figure 1: Single-molecule conductance measurements. ( a ) Schematic of the mechanically controllable break junction (MCBJ) measurements during the photo-conversion of dihydroazulene under the in situ ultraviolet (UV) irradiation. The solution contains dihydroazulene ( dha- 6 ) and vinylheptafulvene ( vhf ). ( b ) Typical individual conductance–distance traces recorded in break junction measurements; blue for the dha- 6 junction and red for the vhf junction. The applied bias potential is 100 mV. ( c ) 2D conductance–displacement histogram constructed from 1,000 conductance–distance traces, the conductance region 10 −3.0 ∼ 10 −4.5 G 0 is defined as region 1, and the conductance region 10 −4.5 ∼ 10 −6.0 G 0 is defined as region 2. Linear scaling is applied for the colour bar. ( d ) 2D covariance histogram constructed from 1,000 conductance–distance traces. Full size image To probe the photo-conversion process of dha- 6 , we introduced the in situ UV irradiation system to the MCBJ setup. In the initial state ( dha- 6 solution without UV irradiation), all the molecular junctions are formed by trapping the dha- 6 into the nanogaps ( dha- 6 junction). The conductance traces show the plateau in the range 10 −3.0 ∼ 10 −4.5 G 0 , and the maximum conductance peak around 10 −3.7±0.1 G 0 is obtained by a Gaussian fitting of the constructed 1D histogram. With UV irradiation (365 nm), the dha- 6 undergoes a ring-opening process of the five-membered ring to form vhf . Thus, both dha- 6 and vhf exist in the solution simultaneously. During the conductance measurements, two kinds of conductance traces are observed, one with a plateau around 10 −3.0 ∼ 10 −4.5 G 0 (marked as region 1) assigned to dha- 6 junction (blue traces) and the other with a plateau around 10 −4.5 ∼ 10 −6 G 0 (marked as region 2), which is ascribed to vhf junctions. The 1D conductance histogram is plotted in Fig. 1b (right part), showing two distinct conductance peaks. The constructed 2D conductance–displacement histogram ( Fig. 1c ) also shows two well-distinguished conductance features with more than one order of magnitude (1.4) conductance difference between them and almost the same plateau length. Moreover, we analysed the correlation between these two kinds of conductance traces by compiling the 2D covariance histogram in Fig. 1d (ref. 21 ). The significant anti-correlation in the intersection of region 1 and region 2 indicates that the molecular junction is constructed either by dha- 6 or vhf for each stretching cycle. Therefore, we can extract each type of conductance trace to quantitatively determine the percentages of dha- 6 and vhf in solution. Photo-thermal reaction kinetics To further investigate the photoreaction process of the dha- 6 , we studied the reaction kinetics with in situ UV irradiation by statistical analysis of the percentage of dha- 6 as a function of time. Based on the anti-correlation between dha- 6 junction and vhf junction mentioned above, the ratio of dha- 6 /vhf or the content of each component ( dha- 6 or vhf ) could be determined from counting the traces presenting each conductance character, although there are around 5–10% traces exhibiting direct tunnelling without forming a molecular junction. 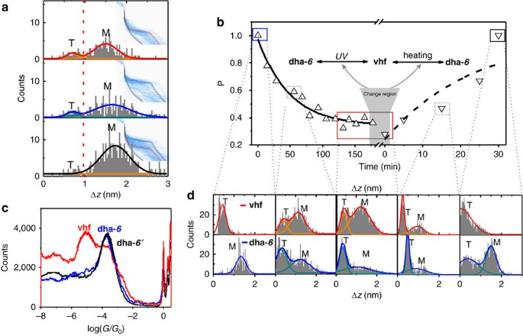Figure 2: Photo-thermal reaction kinetics. (a) The typical relative displacement distributions of MCBJ conductance measurements with thein situUV irradiation (30 min). The conductance regions of the top, middle and below section are 10−4.5∼10−6G0(vhf), 10−3.0∼10−4.5G0(dha-6) and whole region of 10−3.0∼10−6G0, respectively. The Gaussian fitting is used to determine the area ratio of M and T, in which the peak marked as T is ascribed to the tunneling traces and M is for the molecular junction traces. (b) Thedha-6percent versus the reaction time. The upright triangle presents the data points determined from thein situUV irradiation process, and fitted with the exponential function,P=P0+A× exp (−R0t) (black solid curve), to calculate the time decay constant. The inverted triangle shows the data points from theex situheating process, and is fitted withP=1−(1−P0) × exp(−R0t) (black dashed curve). (c) One-dimensional (1D) conductance histogram from different states. Blue is for the initialdha-6state marked with blue solid box inb; red is for the state afterin situUV irradiation for 120 min, marked as red solid box inb; black is from the state after the heating for 30 min connected with the state marked as black solid box inb. The overlapping of blue and black curves suggests a highly reversibledha-6←vhfconversion. Due to the limited time for recording during thein situUV-MCBJ measurements, the numbers of conductance curves for the statistical analysis are limited to around 500. (d) Plateau distribution of the break junctions from different reaction times connected tob. The conductance region ofvhfis 10−4.5∼10−6G0, and that ofdha-6is 10−3.0∼10−4.5G0. Figure 2a shows the typical relative displacement distributions of conductance from MCBJ measurements with in situ UV irradiation (30 min). To determine the time-dependent junction evolution, 500 conductance curves are used for the statistical analysis for each time period. Using the conductance range of 10 −3.0 ∼ 10 −4.5 G 0 (region 1) and 10 −4.5 ∼ 10 −6 G 0 (region 2), we are able to construct the relative displacement distribution for dha and vhf , respectively. In the relative displacement distributions [20] shown in Fig. 2a , the Gaussian fitting of the two peak distributions suggests that the traces with molecular junction (marked with M) are typically longer than 1 nm, while the tunnelling traces without molecular plateau are typically at around 0.5 nm (marked with T). In this way, we could determine the peak area ratio of dha- 6 or vhf junctions from the Gaussian fitting of displacement distribution of all conductance traces including the dha- 6 (or vhf ) junction traces and tunnelling traces (see Supplementary Fig. 22 for more details). Therefore, the percentage of dha- 6 junctions in all molecular junctions could be determined for the further kinetics analysis. Figure 2: Photo-thermal reaction kinetics. ( a ) The typical relative displacement distributions of MCBJ conductance measurements with the in situ UV irradiation (30 min). The conductance regions of the top, middle and below section are 10 −4.5 ∼ 10 −6 G 0 ( vhf ), 10 −3.0 ∼ 10 −4.5 G 0 ( dha- 6 ) and whole region of 10 −3.0 ∼ 10 −6 G 0 , respectively. The Gaussian fitting is used to determine the area ratio of M and T, in which the peak marked as T is ascribed to the tunneling traces and M is for the molecular junction traces. ( b ) The dha- 6 percent versus the reaction time. The upright triangle presents the data points determined from the in situ UV irradiation process, and fitted with the exponential function, P = P 0 + A × exp (− R 0 t ) (black solid curve), to calculate the time decay constant. The inverted triangle shows the data points from the ex situ heating process, and is fitted with P =1−(1− P 0 ) × exp(− R 0 t ) (black dashed curve). ( c ) One-dimensional (1D) conductance histogram from different states. Blue is for the initial dha- 6 state marked with blue solid box in b ; red is for the state after in situ UV irradiation for 120 min, marked as red solid box in b ; black is from the state after the heating for 30 min connected with the state marked as black solid box in b . The overlapping of blue and black curves suggests a highly reversible dha- 6 ← vhf conversion. Due to the limited time for recording during the in situ UV-MCBJ measurements, the numbers of conductance curves for the statistical analysis are limited to around 500. ( d ) Plateau distribution of the break junctions from different reaction times connected to b . The conductance region of vhf is 10 −4.5 ∼ 10 −6 G 0 , and that of dha- 6 is 10 −3.0 ∼ 10 −4.5 G 0 . Full size image We use the combination of the in situ UV irradiation and conductance measurements to investigate the photo-conversion kinetics. The typical stretching distance distributions are presented in Fig. 2d , which are constructed from different states during the conversion process. The percentage of dha- 6 , along with the irradiation time, is plotted in Fig. 2b , showing that the vhf content reached saturation after 120 min of UV irradiation. The data (upright triangles) were fitted with the exponential function, P = P 0 + A × exp(− R 0 t ), where P 0 is the final value of the percentage, R 0 is the decay constant of the best-fit curve with units of time −1 used for the calculation of time constant by taking the inverse. Therefore, the time constant for dha- 6 → vhf photoreaction is calculated as 45±5 min, which is higher than the previous results in the solution (less than 5 min) [22] , [23] . Two factors could be responsible for the longer time to equilibrate. Firstly, during the UV irradiation, heating caused by the light is inevitable, which leads to the back reaction ( vhf → dha- 6 ). More importantly, in the molecular junction, a localized surface plasmon resonance will form in nano-gaps (1.5–3 nm) between two Au electrodes under bias potential, leading to a large buildup of photon intensity and high concentration of energetic electrons [11] , [24] . During the in situ UV-MCBJ measurements, the localized surface plasmon resonance excitation effect could compete with the absorption of the photon from the irradiation to accelerate the back reaction. Figure 2b also illustrates that there is no complete conversion from dha- 6 to vhf , that is, we see the decay curve plateau at just under 40% dha- 6 . We therefore speculate that the heating effect from irradiation and plasmon non-radiative decay must increase the back reaction rate under the in situ UV-MCBJ measurements. A consequence of this is that longer irradiation cannot further decrease the percentage of dha- 6 . It also illustrates that we could not obtain the complete conversion from dha- 6 to vhf . Therefore, the heating effect from irradiation and plasmon non-radiative decay could increase the back reaction rate under the in situ UV-MCBJ measurements. It is also confirmed by the experiments with longer time of UV irradiation ( Supplementary Fig. 23 ). To understand the reversible ring-closing process, the ex situ heating of ∼ 60 °C was applied. As plotted in Fig. 2b (inverted triangle), an increasing percentage of dha- 6 with heating time was observed and the vhf fully switched back to dha- 6 (noted as dha- 6 ′ below for clarity) in 30 min. Furthermore, the function of P =1−(1− P 0 ) × exp(− R 0 t ) was applied for the fitting of the thermal process, and the disagreement between the fitting and the experiments suggests that the constraints of the junction may alter the kinetics of the back reaction. The 1D histograms from three states, the initial dha- 6 , vhf after in situ UV irradiation for 120 min, and the dha- 6 ′ after heating 30 min from vhf state, are constructed and displayed in Fig. 2c . It is shown that the conductance peak of dha- 6 ′ overlaps perfectly with dha- 6 , suggesting a highly reversible dha- 6 ← vhf conversion. Photo/thermal conversion of the isomer For the conversion of dha- 6 ← vhf, the reversible switching cycles are performed sequentially. We demonstrate that there is no significant conversion attenuation in conductance ratio; thus, G dha- 6 / G vhf remained approximately 1.4, as shown in Fig. 3a . Therefore, dha- 6 ← vhf can be considered as a highly promising single-molecule switch. However, the conversion ratio of dha- 6 shows slight attenuation from the analysis of plateau distribution, i.e., we see slightly less dha- 6 after every switching cycle. This may be due to the heat accumulation in the nano-gap regime, which significantly shifts the reaction equilibrium of the dha- 6 ← vhf conversion. Together, these two results suggest that while two clear, reversible conductance states are observable at the single-molecule level, incomplete conversion might complicate the operation of a device utilizing an ensemble of molecules, and further work is required to optimize the percentage conversion in a junction. 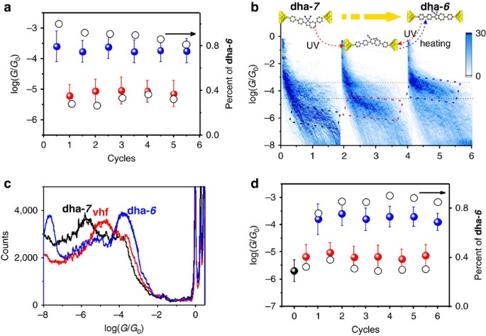Figure 3: Photo/thermal conversion of the isomer. (a) Plot of reversible conversion ofdha-6←vhfin six cycles. The solid circle means the conductance, related to left scale, while the hollow circle is the percentage ofdha-6, related to right scale. (b) Schematic and 2D conductance–displacement histograms for the conversion ofdha-7with the treatments by UV irradiation and heating. (c) One-dimensional (1D) conductance histogram from different states. The black is from the initialdha-7state, the red is for the state after UV irradiation tovhfand the blue is from the conductance measurements for solution after heating process. (d) Plot of conductance switch cycles starting fromdha-7. The error bars of the conductance are determined from the conductance analysis based on Gaussian Function (s.d.). The solid circle means the conductance, related to left scale, while the hollow circle is the percentage ofdha-6, related to right scale. Figure 3: Photo/thermal conversion of the isomer. ( a ) Plot of reversible conversion of dha- 6 ← vhf in six cycles. The solid circle means the conductance, related to left scale, while the hollow circle is the percentage of dha- 6 , related to right scale. ( b ) Schematic and 2D conductance–displacement histograms for the conversion of dha- 7 with the treatments by UV irradiation and heating. ( c ) One-dimensional (1D) conductance histogram from different states. The black is from the initial dha- 7 state, the red is for the state after UV irradiation to vhf and the blue is from the conductance measurements for solution after heating process. ( d ) Plot of conductance switch cycles starting from dha- 7 . The error bars of the conductance are determined from the conductance analysis based on Gaussian Function (s.d.). The solid circle means the conductance, related to left scale, while the hollow circle is the percentage of dha- 6 , related to right scale. Full size image As introduced in Fig. 4 , switching between vhf and dha- 6 is not the only possible reaction for this system as the reverse reaction can, in principle, lead to dha- 7 . As we did not see evidence of this conversion when starting from dha- 6 , dha- 7 was prepared by chemical synthesis [25] and taken as the precursor. During the conductance measurements, the operations of UV irradiation and thermal heating were also applied to dha- 7 . The 2D conductance–displacement and 1D conductance histograms from one photo-thermal cycle are shown in Figs 3b-3c . The conductance measurements demonstrated that the conductance of dha- 7 (10 −5.8±0.1 G 0 ) is lower than that of dha- 6 , and it is also even lower than that of the ring-opened vhf state. More interestingly, in the case of the dha- 7 , after one photo/heating cycle, we only obtained one conductance peak, at G =10 −3.7±0.1 G 0 , implying an almost complete conversion back to dha- 6 . Thus we conclude that the isomerization dha- 7 → vhf → dha- 6 occurred during the UV irradiation and heating reaction cycle. As shown in Fig. 3b , the UV irradiation triggers the ring-opening reaction and vhf is formed, followed by equilibration between vhf isomers. During the ring-closing reaction under the thermal heating, however, only dha- 6 is formed. This can be seen in the 2D histogram, which exhibits an intensive conductance cloud around G =10 −3.7±0.1 G 0 , ascribed to dha- 6. After the first complete switching cycle, almost no conductance features of dha- 7 are observed, shown in Fig. 3b (right). Afterwards, six photo-thermal cycles were performed. It was clear that the conductive properties are quite similar with dha- 6 , including the reversibility and switching, as depicted in Fig. 3d . The conductance switched between high conductance ( dha- 6 , 10 −3.7±0.1 G 0 ) and low conductance ( vhf , 10 −5.1±0.1 G 0 ) with ratio of around 25. 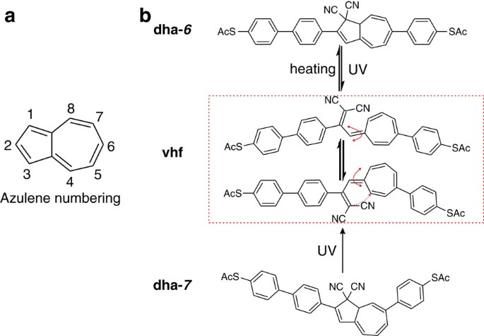Figure 4: The structure of the molecules studied in this work. (a) The numbering used around azulene. (b) The molecular structures of the systems studied and the conversions observed in junction. The system can switch amongdha-6,vhfanddha-7, where the numbers 6 and 7 refer to the position of anchoring group substitution in the seven-membered ring ofdha. Figure 4: The structure of the molecules studied in this work. ( a ) The numbering used around azulene. ( b ) The molecular structures of the systems studied and the conversions observed in junction. The system can switch among dha- 6 , vhf and dha- 7 , where the numbers 6 and 7 refer to the position of anchoring group substitution in the seven-membered ring of dha . Full size image While complete conversion of dha- 7 to dha- 6 was observed in the junction, which is probably promoted by a more favorable anchoring configuration of dha- 6 or by a difference in the vhf to dha transition state dipole moments ( vide infra ), no such preference for dha- 6 has been observed in solution. Irradiating a solution of dha- 7 in CD 3 CN at 365 nm for ca. 2 h gave a mixture of E / Z isomeric vhf s according to 1 H-NMR spectroscopy (see Supplementary Information). After 2 days in the dark, the vhf s underwent conversion to a mixture of dha- 7 and dha- 6 in a ratio of 4:3. Isomerization was also confirmed by UV–Vis absorption spectra in solution. Thus, subjecting a pristine sample of either dha- 6 ( λ max 393 nm) or dha- 7 ( λ max 372 nm) to one opening-closure cycle in CH 3 CN gave a mixture of isomers indicated by an intermediate absorption maximum at ca. 380 nm. Density functional theory calculations In an effort to gain insight into the reaction kinetics of the switch and the discrepancy between the behaviours in solution and junction in regard to isomerization, we investigated the potential energy surface connecting the vhf and dha isomers using density functional theory calculations. Information on the details is given in the Supplementary Information. The energy profile of the system (employing acetonitrile as solvent) is shown in Fig. 5a . We find that the free energies of dha- 6 and dha- 7 are very similar which is in good agreement with the outcome from experimental solution studies. The vhf isomers are connected to the dha species via transition states with similar energy barriers exceeding 20 kcal mol −1 . The barriers for conversion between vhf isomers are much lower and we can therefore assume chemical equilibrium between the vhf isomers at all times in solution. Since the conversion from vhf to either dha is thermally activated, it is highly sensitive to the barrier heights. Any asymmetry in the barrier height would therefore lead to the promotion of one dha isomer over the other before chemical equilibrium is reached. The agreement between the experimental and theoretical solution studies suggests that it is something peculiar to the junction environment that leads to the switching asymmetry. One notable difference between metal electrodes and solution is the ability of electrodes to polarize and screen charges, thereby stabilizing polar/charged systems. We find that the dipole moment of the transition state of Z -vhf → dha- 7 is slightly smaller than for E -vhf→ dha- 6 . We therefore speculate that screening of the dipole moment from electrons in the leads or enhanced electric fields associated with the Au nano-gap might promote the local formation of dha- 6 relative to dha- 7 . Since spontaneous ring-opening should occur at time-scales much longer than the experiment, this would explain why dha- 6 is preferentially observed in the break-junction experiment. 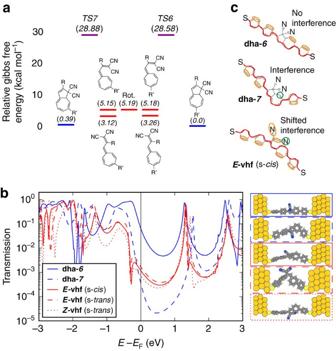Figure 5: Calculated energy and transport properties. (a) Potential free energy profile of thedhaandvhfspecies in acetonitrile solution. (b) Calculated transmissions for structures are shown on the right. Zero-bias conductance indicatesG(dha-6)>G(vhf)>G(dha-7), in agreement with experiment. (c) Example diagrams. No interference is expected at the Fermi energy fordha-6because all diagrams without onsite loops have the same sign. Fordha-7, all diagrams contain the same onsite loop so destructive interference is expected at the Fermi energy. Forvhf, diagrams with onsite loops on N shift the interference away from the Fermi energy. Figure 5: Calculated energy and transport properties. ( a ) Potential free energy profile of the dha and vhf species in acetonitrile solution. ( b ) Calculated transmissions for structures are shown on the right. Zero-bias conductance indicates G ( dha- 6 )> G ( vhf )> G ( dha- 7 ), in agreement with experiment. ( c ) Example diagrams. No interference is expected at the Fermi energy for dha- 6 because all diagrams without onsite loops have the same sign. For dha- 7 , all diagrams contain the same onsite loop so destructive interference is expected at the Fermi energy. For vhf , diagrams with onsite loops on N shift the interference away from the Fermi energy. Full size image For comparing the energies of the two molecules dha- 6 and dha- 7 when placed in a junction (ensuring interactions between molecule and metal leads), we performed combined QM/MM calculations [26] using the program Dalton QCP [27] . The gold electrodes are built as two hemispheres from a fcc unit cell and described using molecular mechanics. Each gold cluster consists of 262 Au atoms, where each gold atom is assigned a polarizability of 31.04 a.u. The molecule faces the [111] surface with the axis through the two sulfur atoms oriented perpendicular to the gold surface. The density functional theory geometry-optimized molecules were inserted between the two gold clusters and then single point energy calculations were performed (CAM-B3LYP//cc-pVDZ). Interestingly, we find that dha- 6 is more stable than dha- 7 by 3.04 kcal mol −1 in the junction, while the difference was only 0.39 kcal mol −1 for the molecules in solution (acetonitrile). A smaller difference between the reactive s- cis Z -vhf and s- cis E -vhf isomers was obtained, with the Z -vhf being 0.72 kcal mol −1 more stable than the E -vhf . Although the slightly more energetic E -vhf is the precursor for dha- 6 , it pays off overall from a thermodynamic point of view to form dha- 6 in the junction. We were not able to perform reliable TS calculations in the junction in order to ascertain whether the kinetics of ring closure also agrees with experiment. Nevertheless, we have previously observed that the larger the dha − vhf energy difference, the faster is the vhf -to- dha conversion [27] , [28] , [29] . Despite the chemical similarities of dha- 6 , vhf and dha- 7 , their calculated transport properties are vastly different and followed the trend dha- 6 > vhf > dha- 7 in the experiments. A theoretical analysis using a diagrammatic approach first used by Markussen et al . [30] , [31] combined with density functional theory transport calculations shows that dha- 6 has the highest conductance because it is almost planar and does not show destructive interference ( Fig. 5b ). Conversely, dha- 7 and vhf are bent and show destructive interference. The difference between these two systems results from the different energies at which the interference feature occurs. The diagrammatic description predicts no destructive interference for dha- 6 because it is possible to pair up all the non-traversed π-orbitals along the path connecting the electrodes for these molecules. However, this is not possible for dha- 7 and vhf as illustrated in Fig. 5c . In dha- 7 , the anchoring group is placed at C7, which causes significant deviation of the π -system from planarity as also confirmed by X-ray crystallographic analysis ( Fig. 6 ). Moreover, the cyano groups are electronically decoupled from the rest of the π-system by saturated bonds and destructive interference therefore occurs in the middle of the band gap. This decoupling is not present in vhf and the anti-resonance is therefore shifted away from the middle of the band gap due to the electron-accepting character of CN. The calculated features of dha- 6 and dha- 7 are in line with their different optical properties determined experimentally ( vide supra ): dha- 6 exhibits a red-shifted longest-wavelength absorption maximum relative to dha- 7 . 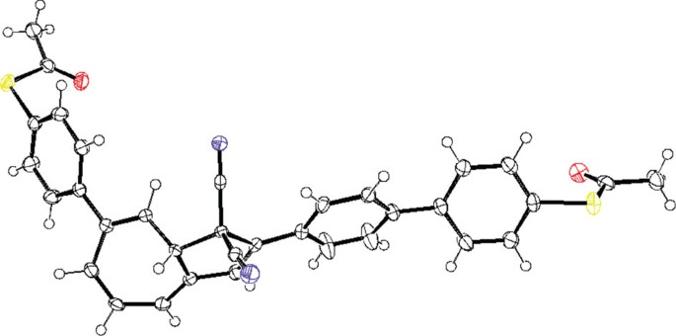Figure 6: X-Ray crystal structure. Molecular structure ofdha-7with displacement ellipsoids of 50% for non H-atoms (CCDC 1501743); red: oxygen; yellow: sulfur; blue: nitrogen. Crystals were grown from dichloromethane and heptane. Figure 6: X-Ray crystal structure. Molecular structure of dha- 7 with displacement ellipsoids of 50% for non H-atoms (CCDC 1501743); red: oxygen; yellow: sulfur; blue: nitrogen. Crystals were grown from dichloromethane and heptane. Full size image To conclude, we have developed an approach to detect the photo-thermal reaction of dha / vhf system using the single-molecule break junction technique. We have demonstrated that this technique is able to track the photo-thermal reaction, and to evaluate the reversibility and multiple switching possibilities during the reaction using the well-distinguished conductance states of single-molecule dha / vhf junctions. The combined transport calculations suggest that these distinct conductance states were ascribed to the introduction and shifting of interference features in the molecular transmission. More importantly, beyond simply the application as a molecular switch, this study raises questions about tuning reaction kinetics, barriers and ultimately product ratios in the novel environment of molecular junctions. While we saw clear and reversible switching, the product ratio obtained does not correspond with that observed in solution studies. It remains a question for future work whether the product ratios can be further tuned by junction engineering or if this principle can be employed to tune product ratios for other reactions. Single-molecule conductance measurement Conductance measurements were performed using the MCBJ technique with a home-built MCBJ setup [19] , [20] . To perform the conductance measurement, the solution contains 0.2 mM target molecules in mixture solvent of THF:Mesitylene (TMB)=1:4. A blank experiment of solvent without target molecule is presented in Supplementary Fig. 21 . UV irradiation and heating experiment To have the in situ UV irradiation experiment, one UV LED at 365 nm is built with the power of 300 μW cm −2 . The home-built UV LED was put on the top of the solution with a distance of ∼ 1 cm. As for the photo-conversion kinetic studies, the UV LED were turned on during the conductance measurements. In the ex situ heating process, the solution was put in a water bath with constant temperature (65 °C). After setting waiting time (0, 5, 15, 25 and 30 min), we took 200 μl solution into the liquid cell of MCBJ for conductance measurements. Synthesis and characterization Synthesis and NMR characterization are provided in Supplementary Figs 1–5 and Supplementary Note 1 . UV–Vis and NMR spectroscopic studies in solution are provided in Supplementary Figs 6–10 and Supplementary Note 2 . Details on the theoretical work are provided in Supplementary Figs 11–20 , Supplementary Table 1 and Supplementary Notes 3–6 . Data availability The X-ray crystallographic coordinates for the structure reported in this article have been deposited at the Cambridge Crystallographic Data Centre (CCDC), under deposition number CCDC 1501743. These data can be obtained free of charge from The Cambridge Crystallographic Data Centre via www.ccdc.cam.ac.uk/data_request/cif . The data that support the findings of this study are available from the corresponding author upon reasonable request. How to cite this article: Huang, C. et al . Single-molecule detection of dihydroazulene photo-thermal reaction using break junction technique. Nat. Commun. 8, 15436 doi: 10.1038/ncomms15436 (2017). Publisher’s note : Springer Nature remains neutral with regard to jurisdictional claims in published maps and institutional affiliations.